Structure and mechanism of action of the hydroxy–aryl–aldehyde class of IRE1 endoribonuclease inhibitors Endoplasmic reticulum (ER) stress activates the unfolded protein response and its dysfunction is linked to multiple diseases. The stress transducer IRE1α is a transmembrane kinase endoribonuclease (RNase) that cleaves mRNA substrates to re-establish ER homeostasis. Aromatic ring systems containing hydroxy–aldehyde moieties, termed hydroxy–aryl–aldehydes (HAA), selectively inhibit IRE1α RNase and thus represent a novel chemical series for therapeutic development. We solved crystal structures of murine IRE1α in complex with three HAA inhibitors. HAA inhibitors engage a shallow pocket at the RNase-active site through pi-stacking interactions with His910 and Phe889, an essential Schiff base with Lys907 and a hydrogen bond with Tyr892. Structure–activity studies and mutational analysis of contact residues define the optimal chemical space of inhibitors and validate the inhibitor-binding site. These studies lay the foundation for understanding both the biochemical and cellular functions of IRE1α using small molecule inhibitors and suggest new avenues for inhibitor design. Endoplasmic reticulum (ER) stress and the resulting unfolded protein response (UPR) have gained significant interest as an area in which targeted molecules may have extensive therapeutic overlap in divergent disease types including neurodegeneration, inflammation, metabolic syndromes and cancer [1] , [2] . The ER is a large intracellular compartment responsible for the production of secreted and cell surface proteins as well as cellular lipid biosynthesis and membrane generation. The ER is physically connected to both the nucleus and the mitochondria and is fundamentally integrated with global cellular regulatory networks and metabolism. Protein folding, membrane and nutrient perturbations within the ER, arising from exogenous or internal stresses, induce the UPR [3] . This cellular signalling response serves to alleviate the imposing stress and corrects the imbalance to restore normal cellular homeostasis. However, accumulating evidence suggests that the UPR, when chronically activated due to a myriad of stimuli, may be pathological resulting in inflammation, cell death or conversely may be exploited by cancer cells to ensure survival [1] , [3] , [4] , [5] . The three major arms of the fully integrated UPR include PERK (pancreatic eIF2alpha kinase), ATF6 (activating transcription factor 6) and IRE1 (inositol-requiring enzyme 1), which function as a finely tuned triad. All three arms have overlapping yet distinct responsibilities and regulate a plethora of downstream genes [3] . PERK, an ER-resident transmembrane eIF-2α kinase, halts translation [6] to induce transcriptional programs via non-conventional translation of ATF4, which results in both pro-life and pro-death outcomes [7] . During ER stress, ATF6 is translocated to the Golgi where it undergoes proteolysis at the membrane releasing it to the nucleus [8] where it transactivates genes required for the UPR [9] . IRE1, the most conserved arm of the UPR, is a unique ER transmembrane fused dual kinase-endoribonuclease [10] that directly regulates HAC1 in yeast or its metazoan orthologue XBP1 (refs 3 , 4 ). Fungi possess a single isoform of IRE1, while higher eukaryotes generally possess two isoforms denoted IRE1α and β. The endoribonuclease (RNase) domain of IRE1, which appears unique to eukaryotes [11] , [12] , [13] , [14] , [15] , is found in only one other paralogue, RNase L [16] , an enzyme involved in innate immunity in vertebrates [17] . UPR signalling initiates from the IRE1 luminal domain, which senses the accumulation of unfolded protein, proceeds by dimerization and oligomerization to activate the cytoplasmic auto-kinase activity [18] , [19] and in turn RNase activity [10] , [20] . In metazoan organisms, selective cleavage of dual stem loops within the XBP1 mRNA ensues and a 26-nucleotide intron is removed [21] , [22] , [23] . The two exon ends are then ligated by an unknown process [24] allowing the spliced XBP1 ( XBP1 s) transcript to be translated into a functional transcription factor. XBP1s directs the transcription of chaperones, ERAD (ER-associated protein degradation) components and other targets involved in ER expansion, phospholipid synthesis and general homeostasis [25] . Combined, the downstream activities of the XBP1s transcriptional network can enforce specialized cellular functions such as antibody secretion in plasma cells [26] . In addition to XBP1 mRNA, IRE1 also cleaves a selected set of ER-targeted mRNAs [27] . This process, termed RIDD (regulated IRE1-dependent decay) [28] , attempts to rapidly decrease the secretory load during ER stress; however, little is known about its physiological significance [28] , [29] . Recent evidence suggests that IRE1α can be activated in response to specific signalling events independent of the UPR, which have cell type- or organ-specific functions and can be dependent [30] or independent of XBP1 (refs 31 , 32 ). The kinetics of IRE1α signalling usually follows a rapid on–off response where activation is followed by rapid deactivation [33] , which can have longer-term consequence [34] . This is achieved by yeast IRE1 through dephosphorylation [35] or hyperphosphorylation [36] of the kinase. Small molecule modulators of IRE1 kinase and RNase functions have been reported with distinct mechanisms of action reflecting the engagement of three physically distinct binding sites. Kinase domain active site binders inhibit kinase output by virtue of ATP competition and paradoxically can either potentiate [37] , [38] or inhibit [39] RNase output depending on the underlying chemotype. The structural basis for their differential effect on RNase function has not been resolved since X-ray crystal structures of RNase inhibitors bound to the IRE1 kinase domain specifically are lacking. Quercetin, representative of a second class of modulators, marginally influences the kinase output of yeast IRE1 while potently enhancing RNase output by promoting molecular dimerization through engagement of a composite binding pocket at the enzyme–dimer interface [40] . Salicylaldehyde derivatives represent a third class of modulators that potently, reversibly and selectively inhibit IRE1 RNase activity [41] , with weak effects on protein kinase function. Additional compounds using the adjacent hydroxy–aldehyde motif and dual-ring biphenyl (WO 2008/154484 A1), naphthalene (WO 2008/154484 A1; WO 2011/056744 A1) and coumarin (WO 2011/127070 A2) aromatic systems, which we collectively refer to as hydroxy–aryl–aldehydes (HAA), were also found to be potent IRE1 RNase inhibitors [42] , [43] , [44] . Notably, a combination of methods including chemical modification of the protein/HAA inhibitor complex demonstrated that the aldehyde forms a reversible Schiff base with lysine 907 in the active site region of the RNase domain [43] . These findings were surprising and offered hope for the selective and potent targeting of IRE1 where RNase-active sites in general have made poor drug targets as they possess hydrophobic pockets that are shallow or non-existent due to a requirement for extensive interactions with the RNA phosphodiester backbone. Here we uncover the structural basis for HAA inhibitor mechanism of action through a detailed X-ray crystallographic study of three members, representative of two different chemical scaffolds, in complex with murine IRE1α (referred here generally as IRE1α). These structures and follow-up analyses allow for a rationalization of structure–activity relationships (SARs) and suggest avenues for future optimization. Co-crystallization and characterization of HAA inhibitors To discern the mechanism of action of the HAA class of IRE1-specific endoribonuclease inhibitors, we pursued X-ray crystallographic analyses of HAA members in complex with the dual catalytic region of IRE1. In an extensive screening campaign, sampling combinations of HAA inhibitors with nucleotides, protein kinase inhibitors and IRE1α orthologues (yeast, zebrafish, human and mouse) with different N-terminal domain boundaries and phosphorylation states, we obtained suitable co-crystals for three HAA inhibitors, namely, MKC9989, OICR464 and OICR573 (see Fig. 1a for chemical structures and substituent numbering schemes). Each was obtained in complex with Mg 2+ /ADP and an auto-phosphorylated minimal dual catalytic domain fragment of murine IRE1α encompassing residues 549–977. 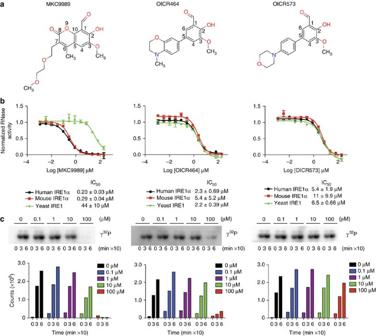Figure 1: Functional characterization of HAA inhibitors solved in complex with IRE1α. (a) Chemical structure and substituent numbering scheme of HAA inhibitors. (b) Inhibition of IRE1 RNase activity by HAA inhibitors using a real-time fluorescence readout assay. IC50s derived from fitted profiles represent the mean±s.d.,n=6 (three experiments performed in duplicate) for murine IRE1α and yeast IRE1 andn=4 (two experiments performed in duplicate) for human IRE1α. Shown are representative profiles for one experiment performed in duplicate. (c) Inhibition of IRE1α auto-kinase activity by HAA inhibitors. The crystals diffracted at 2.9, 3.0 and 3.4 Å resolution, respectively, and the co-structures were solved by molecular replacement using the human IRE1α crystal structure as a search model (see Methods for experimental details and Table 1 for data collection and refinement statistics). Figure 1: Functional characterization of HAA inhibitors solved in complex with IRE1α. ( a ) Chemical structure and substituent numbering scheme of HAA inhibitors. ( b ) Inhibition of IRE1 RNase activity by HAA inhibitors using a real-time fluorescence readout assay. IC 50 s derived from fitted profiles represent the mean±s.d., n =6 (three experiments performed in duplicate) for murine IRE1α and yeast IRE1 and n =4 (two experiments performed in duplicate) for human IRE1α. Shown are representative profiles for one experiment performed in duplicate. ( c ) Inhibition of IRE1α auto-kinase activity by HAA inhibitors. Full size image Table 1 Data collection and refinement statistics. Full size table MKC9989, OICR464 and OICR573 inhibitors visualized in IRE1α co-structures potently inhibited the RNase activity of murine and human IRE1α, and to a lesser degree yeast IRE1 in the case of MKC9989 in vitro with IC 50 s ranging from 0.23 to 44 μM ( Fig. 1b ). In contrast, the same inhibitors had no effect or weakly inhibited the auto-kinase activity of IRE1α at the highest concentrations tested (IC 50 s>>10 μM) ( Fig. 1c ). In the case of OICR464 and OICR573 (and to a lesser extent MKC9989), inhibitor potency showed a significant dependency on pre-incubation time with IRE1α ( Supplementary Fig. 1 ). This may reflect differences in the reactivity of the aldehyde group in each HAA scaffold required to support formation of a Schiff base interaction with Lys907. At 10 μM concentration, MKC9989 completely inhibited both basal and thapsigargin-induced splicing of XBP1 mRNA ( Fig. 2a ). These effects were observed even in cells pre-treated with thapsigargin, indicating that MKC9989 can fully reverse the onset of XPB1 splicing after the UPR is initiated. In parallel analyses, MKC9989 markedly stabilized the RIDD target CD59 mRNA [45] when co-administered with thapsigargin relative to thapsigargin treatment alone and modestly increased levels of CD59 mRNA in non-stressed cells, the latter likely reflecting the inhibition of baseline RIDD activity. In contrast to the effects on XBP1 splicing, MKC9989 moderately stabilized CD59 levels when administered 2 h post treatment with thapsigargin. Finally, the potency of MKC9989 against the splicing of XBP1 mRNA (EC 50 =0.33 μM) was comparable to its potency against RNA cleavage in vitro ( Fig. 1b ). These functional properties in total suggested that the MKC9989, OICR464 and OICR573 X-ray co-structures could help illuminate the mechanism of action of the HAA class of inhibitors in vitro and in cells. 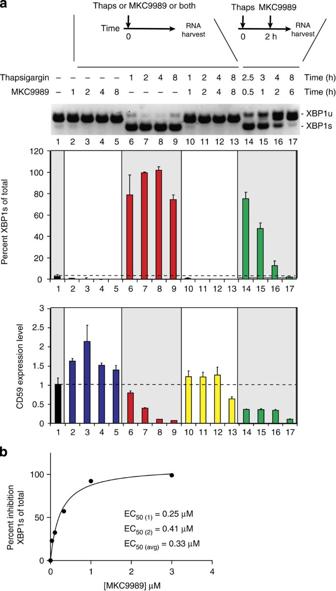Figure 2: Inhibition of IRE1α function by MKC9989 in human RPMI 8226 plasmacytoma cells. (a) Time course analysis of MKC9989 inhibitory function onXBP1splicing: reverse transcription PCR PAGE analysis (top) and quantification (middle) of XBP1-spliced products from three independent experiments shown as±s.e.m. Quantification ofCD59transcript levels from the same RNA samples (bottom). (b) Dose-response analysis of MKC9989 treatment onXBP1splicing in human RPMI 8226 plasmacytoma cells. Shown is a representative profile with EC50calculated as the average of two independent experiments. Figure 2: Inhibition of IRE1α function by MKC9989 in human RPMI 8226 plasmacytoma cells. ( a ) Time course analysis of MKC9989 inhibitory function on XBP1 splicing: reverse transcription PCR PAGE analysis (top) and quantification (middle) of XBP1-spliced products from three independent experiments shown as±s.e.m. Quantification of CD59 transcript levels from the same RNA samples (bottom). ( b ) Dose-response analysis of MKC9989 treatment on XBP1 splicing in human RPMI 8226 plasmacytoma cells. Shown is a representative profile with EC 50 calculated as the average of two independent experiments. Full size image Structure overview In all three HAA co-structures, IRE1α crystallized in the same face-to-face dimer configuration adopted by human IRE1α [46] , and not the back-to-back dimer or oligomer configuration adopted by yeast IRE1 (refs 11 , 37 ) ( Fig. 3a ). This conservation lends further support to the notion that the face-to-face dimer configuration is a functionally relevant conformation for IRE1α and raises the question why the human and mouse IRE1 orthologues did not adopt the back-to-back dimer configuration reflective of the ‘RNase-active’ state. Each protomer of IRE1α consisted of a bilobal protein kinase domain rigidly fused through the kinase C-lobe to an α-helical RNase domain. All IRE1α protomers in each co-structure displayed unambiguous density for Mg 2+ /ADP in the catalytic cleft of the kinase domain ( Supplementary Fig. 2a ). Minimally, one IRE1α protomer per co-structure displayed a well-ordered HAA inhibitor engaging the active site of the RNase domain ( Supplementary Fig. 2a,b ). The remaining RNase-active sites were occluded by crystal packing, or weak electron density precluded accurate modelling of the bound inhibitor. IRE1α protomers were well ordered with the exception of ~13 residues at both N and C termini and also within the kinase domain activation segment (residues 719–730). IRE1α protomers were highly similar to each other (r.m.s.d.=0.24 Å 2 over 10 total molecules in the asymmetric unit of the three HAA co-structures), to human IRE1α protomers (Protein Data Bank (PDB) 3P23, r.m.s.d.=1.28 Å 2 ) and to yeast IRE1 protomers (PDB 3LJ0, r.m.s.d.=1.48 Å 2 ). 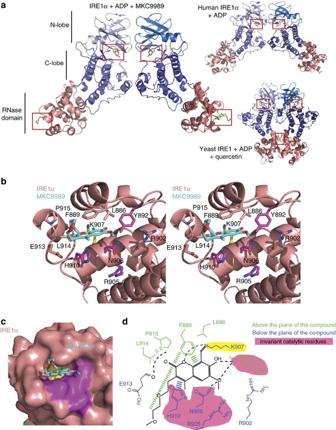Figure 3: Crystal structure of IRE1α bound to MKC9989. (a) Ribbons representation of a face-to-face dimer configuration of IRE1α in complex with Mg2+/ADP and MKC9989. ADP engaging the kinase-active site and MKC9989 engaging the RNase-active site are shown as sticks and highlighted by red boxes. For comparison, the dimer configurations adopted by human IRE1α (PDB 3P23) and yeast IRE1 (PDB 3LJ0) are shown at right. (b) Ribbons’ stereo representation of MKC9989 engaging the RNase-active site of IRE1α. Invariant active site residues, Lys907 and other conserved residues in the binding pocket are coloured purple, yellow and pink, respectively. Lys907 forms a Schiff base to the aldehyde moiety of MKC9989. (c) Zoom in surface view of the IRE1α–MKC9989 complex coloured as inb. (d) Schematic of contact residues and notable interactions mediating MKC9989 binding to IRE1α. Figure 3: Crystal structure of IRE1α bound to MKC9989. ( a ) Ribbons representation of a face-to-face dimer configuration of IRE1α in complex with Mg 2+ /ADP and MKC9989. ADP engaging the kinase-active site and MKC9989 engaging the RNase-active site are shown as sticks and highlighted by red boxes. For comparison, the dimer configurations adopted by human IRE1α (PDB 3P23) and yeast IRE1 (PDB 3LJ0) are shown at right. ( b ) Ribbons’ stereo representation of MKC9989 engaging the RNase-active site of IRE1α. Invariant active site residues, Lys907 and other conserved residues in the binding pocket are coloured purple, yellow and pink, respectively. Lys907 forms a Schiff base to the aldehyde moiety of MKC9989. ( c ) Zoom in surface view of the IRE1α–MKC9989 complex coloured as in b . ( d ) Schematic of contact residues and notable interactions mediating MKC9989 binding to IRE1α. Full size image Binding mode of HAA inhibitors to the RNase domain of IRE1 The structure of the IRE1α RNase domain consisted of nine α-helices (denoted helices α1–α8 and α3′). All three HAA inhibitors shared similar binding modes with a shallow pocket nestled at the nexus of helices α3′, α4 and α5, and lined by the side chains of Glu913, Leu914, Pro915, Phe889, Leu886, Lys907 and Arg902, and the invariant or highly conserved catalytic residues Tyr892, Arg905, Asn906, His910 and Arg902 ( Fig. 3b , Supplementary Fig. 3a,b ). Using the human IRE1α structure (PDB3P23) as a reference for the apo state of the RNase domain, comparison with IRE1α in complex with HAA inhibitors revealed that the HAA-binding pocket was largely preformed ( Supplementary Fig. 3c,d ). Small induced conformational changes consisted of: (1) enforcement of a single rotomer conformer for Asn906 and His910 that enlarged the binding pocket to accommodate the HAA ring structure and (2) a clamping movement of the Phe889 side chain (5.1 Å, Cα to Cα movement) onto the apical surface of the engaged HAA inhibitor. Owing to the overlap with the RNase-active site (three of four invariant active site residues are exploited in the HAA-binding interaction), the HAA-binding pocket is highly conserved ( Supplementary Fig. 3d ) with only a conservative substitution of tyrosine for phenylalanine at position 889 differentiating the binding pocket between fungal and metazoan enzymes ( Supplementary Fig. 4 ). This may explain the general cross-reactivity of HAA inhibitors across IRE1α orthologues tested (yeast, mouse and human) [41] . Conserved interactions across the three co-structures that are predicted to contribute to affinity and specificity of the HAA inhibitor class include: a Schiff base interaction between the HAA aldehyde group and the amine group of Lys907; a hydrogen-bond interaction between the HAA hydroxy group and the side chain of Tyr892; pi-stacking of the Phe889 side chain with the apical surface of the HAA aromatic ring directly harbouring the hydroxy and aldehyde groups; and finally, pi-stacking of the His910 side chain with the basal surface of flanking HAA aromatic rings. All three co-crystallized HAA inhibitors possessed methoxy moieties at a position immediately adjacent to the core hydroxy moiety, and these possess the capacity to hydrogen bond with the side chain of Asn906. Since the methoxy moiety is not a conserved feature of all HAA inhibitors [41] , [42] , [43] , this interaction is not a general feature of the HAA inhibitor-binding mode. Reflecting differences in chemical scaffold and substituent structure, each HAA inhibitor also made a limited number of distinct interactions with the binding pocket on IRE1α that may account for differences in potency. These unique interactions were accommodated in part by plasticity of the binding mode evident by a subtle (~1.5 Å) lateral shift of the single ring core of OICR464 and OICR573 relative to that of the planar fused ring core of MKC9989 ( Supplementary Fig. 3d ). Unique interactions exploited by MKC9989 include: hydrogen bonds between Lys907 and the oxygen heterocycle of the coumarin ring and between Tyr892 and the oxygen atom of the ether moiety at position 3; van der Waals contacts involving the main chain Glu913 and the side chains of Pro915 and Leu914 with the coumarin C=O group; and finally a hydrophobic interaction between the Phe889 side chain and the flexible polyether moiety at position 7 ( Fig. 3b,d ). These inhibitor-specific interactions may account for enhanced potency of MKC9989 relative to OICR464 and OICR573. The aldehyde moiety of HAA inhibitors has been shown to selectively form a reversible Schiff base interaction with Lys907 in the RNase domain and to a lesser degree with Lys599 in the ATP-binding site of the kinase domain, versus 20 other surface-exposed lysine residues within the dual catalytic region of human IRE1α [43] . This reactivity can be rationalized by the position of the Lys907 side chain at the back of a sheltered binding pocket. Due to the clamping action of the Phe889, His910 and Asn906 side chains on either side of the HAA planar ring structure, the Schiff base interaction once formed would be shielded from attack by water. Furthermore, reactivity of the aldehyde towards Lys907 may be enhanced by the electron polarizing hydrogen bond between Tyr892 and the adjacent hydroxy moiety. These features are uniquely supported by the environment around Lys907. The fact that Lys599 displays some reactivity to HAAs may be explained by the sheltered environment of the kinase-active site, which would also shield a Schiff base interaction from attack by water once formed. Using kinase inhibition as a proxy for kinase domain engagement, the interaction of MKC9989 and OICR464 with the kinase-active site Lys599 is ~10- to 100-fold weaker than engagement with Lys907, whereas OICR573 does not appear to engage Lys599 to a detectable degree ( Fig. 1c ). Basis for non-competitive mechanism of action To discern how HAA inhibitors act non-competitively with respect to RNA substrate [41] , [43] while exploiting direct contacts to three of four invariant RNase-active site residues, we modelled a dinucleotide substrate into the active site region of IRE1α bound to MKC9989. As transfer RNA (tRNA) endonuclease, whose X-ray crystal structure was determined in complex with RNA [47] , shares a highly similar active site architecture and inferred catalytic mechanism with IRE1 (ref. 11 ), it provided an instructive template for modelling the IRE1α–RNA substrate–HAA inhibitor complex (see Methods for modelling details). As modelled in Supplementary Fig. 3e , MKC9989 binds immediately opposite to the RNA along an axis linking Asn906, His910 and Arg902 side chains, without overt clashes. His910 has been proposed to act as a general acid that protonates the 5′-OH leaving group, whereas Arg905 and Asn906, the latter supported by a hydrogen-bonding interaction with Tyr892, likely serve to position the scissile phosphate for nucleophilic attack. We reason that subtle changes to the position of three (His910, Asn906 and Tyr892) of these four conserved catalytic residues imposed by HAA inhibitor binding ( Supplementary Fig. 3c ) may be responsible in part for the resultant loss in RNase catalytic function. A more detailed understanding of HAA inhibitor mechanism of action awaits the determination of comparative structures of IRE1α productively bound to RNA and non-productively bound to both RNA and HAA inhibitor. Mutational analysis of the HAA-binding pocket To explore HAA binding determinants on the RNase domain of IRE1α, we mutated the contact residues Phe889, Tyr892, Asn906, His910 and Lys907 in the context of a longer dual catalytic fragment of IRE1α encompassing residues 499–977 ( Fig. 4a ). Consistent with their immediate proximity to the RNase-active site, all five mutations abolished RNase activity against a single hairpin substrate ( Fig. 4b ) while leaving protein kinase activity largely intact ( Fig. 4c ). This limited our ability to infer the effect of mutations on inhibitor binding by the analysis of enzymatic inhibition constants ( K i ). However, using 600-fold higher concentrations of a double hairpin substrate produced in T7 RNA runoff reactions and 10,000-fold higher concentrations of IRE1α, the Lys907Ala and Phe889Ala but not His910Ala, Tyr892Ala and Asn906Leu mutants displayed detectable RNase activity. In contrast to the wild-type enzyme, the Lys907Ala but not the Phe889Ala mutant was insensitive to MKC9989 when assayed under these conditions ( Fig. 4d ). 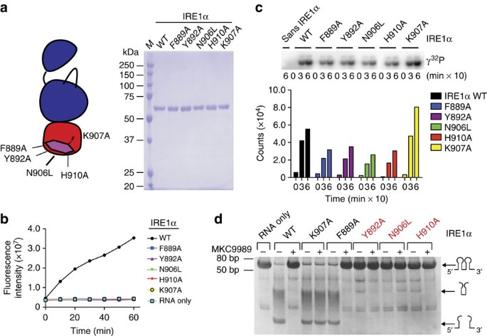Figure 4: SAR of HAA inhibitors and their binding site on IRE1α. (a) Schematic (left) and SDS–PAGE analysis (right) of IRE1α RNase-active site mutants. (b) Effect of RNase-active site mutations on IRE1α RNase function as assessed by a real-time fluorescence readout assay. (c) Effect of RNase-active site mutations on IRE1α kinase function as assessed by auto-kinase activity (phosphor image, top; quantification, bottom). (d) Sensitivity of IRE1α wild-type (WT) and RNase-active site mutants to inhibition of RNase activity by MKC9989 as assessed using a dual-hairpin RNA substrate. Figure 4: SAR of HAA inhibitors and their binding site on IRE1α. ( a ) Schematic (left) and SDS–PAGE analysis (right) of IRE1α RNase-active site mutants. ( b ) Effect of RNase-active site mutations on IRE1α RNase function as assessed by a real-time fluorescence readout assay. ( c ) Effect of RNase-active site mutations on IRE1α kinase function as assessed by auto-kinase activity (phosphor image, top; quantification, bottom). ( d ) Sensitivity of IRE1α wild-type (WT) and RNase-active site mutants to inhibition of RNase activity by MKC9989 as assessed using a dual-hairpin RNA substrate. Full size image Direct binding measurements using microscale thermophoresis revealed a close correlation between IRE1α-binding activity and inhibitor potency, with MKC9989 binding more tightly than OICR464 and OICR573 ( Supplementary Fig. 5a , K d =0.84, 15.9 and 35.2 μM, respectively). Notably, the IRE1α mutations Tyr892Ala ( K d =10 μM), Asn906Leu ( K d =8.9 μM), His910Ala ( K d =5.3 μM) and Phe889Ala ( K d =10.9 μM) perturbed the binding to MKC9989 minimally by 10-fold, while the IRE1α Lys907Ala mutation abolished detectable binding ( Supplementary Fig. 5b ). Together, these results demonstrated the importance of protein interactions visualized in the IRE1α–HAA inhibitor co-structures and highlighted the pre-eminent role for the Schiff base interaction with Lys907 in the HAA inhibitor mechanism of action. Structure–activity relationships To unify our understanding of SAR data as well as validate the binding mode observed in the HAA co-structures, we assembled an HAA analogue series around a naphthalene scaffold [42] (WO 2008/154484 A1; WO 2011/056744 A1) ( Fig. 5 ). This series offered the advantage of more sites around the dual fused ring core for addition of substituents, while the chemical space largely overlaps with the biphenyl and coumarin HAA inhibitors. In keeping with chemical convention, we used a substituent numbering scheme with position 1 corresponding to the aldehyde moiety and position 2 proceeding along the direction of the adjacent hydroxy moiety (MKC3437). Consistent with previous findings for a single aryl ring scaffold [41] , substitution of the aldehyde or hydroxy moieties at positions 1 and 2 were not tolerated (MKC3964 and MKC3820). This likely reflected the importance of the Schiff base interaction with Lys907 and the hydrogen bond interaction with Tyr892, respectively. In accordance with position 3 and 7 facing towards solvent, addition of bulky substituents (MKC3426 and MKC3946) were well tolerated. Substitutions at position 8 were more restrictive owing to the partially buried nature of the interaction site with IRE1α. Addition of a bromine substituent at this position (MKC3987) was favoured relative to hydrogen (IC 50 =0.39 versus 2.2 μM, respectively), while a bulkier methyl-piperizine-carbonyl-phenyl group was disfavoured (MKC4027) (IC 50 =5.7 μM). Like the C=O group of the coumarin scaffold of MKC9989, bromine at position 8 would be accommodated in the narrow confines of the binding site. In contrast, the methyl-piperizine-carbonyl-phenyl group is predicted to sterically clash in the absence of a major shift in inhibitor-binding mode. In summary, these SARs are consistent with the inhibitor-binding mode elucidated by X-ray co-structure and molecular modelling analyses and suggest further avenues for future optimizations. 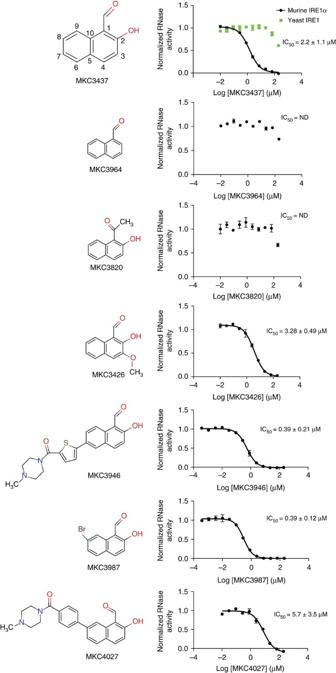Figure 5: SAR analysis of a naphthalene analogue series on IRE1α RNase activity. Shown are analogue structures (left) and RNase inhibition profiles (right). IC50values represent the average forn=4 (two experiments performed in duplicate)±s.d. Displayed profiles represent one experiment performed in duplicate. Substituent numbering scheme and RNase inhibitory activity against yeast IRE1 are shown on top for the minimal naphthalene scaffold MKC3437. Figure 5: SAR analysis of a naphthalene analogue series on IRE1α RNase activity. Shown are analogue structures (left) and RNase inhibition profiles (right). IC 50 values represent the average for n =4 (two experiments performed in duplicate)±s.d. Displayed profiles represent one experiment performed in duplicate. Substituent numbering scheme and RNase inhibitory activity against yeast IRE1 are shown on top for the minimal naphthalene scaffold MKC3437. Full size image ADP as a model for dimer-breaking IRE1α RNase inhibitors Back-to-back dimerization and subsequent polymerization of the fused kinase endoribonuclease catalytic module is required for the RNase activity of yeast IRE1 (ref. 11 ) and presumably all orthologues. The binding of nucleotide and small molecule protein kinase inhibitors to the kinase domain can influence dimer/oligomer formation and as a result RNase activity; ADP, janus kinase (JAK) inhibitor I, cyclin-dependent kinase inhibitor I and APJ (N~2~-1H-benzimidazol-5-YL-N~4~-(3-cyclopropyl-1H-pyrazol-5-YL)pyrimidine-2,4-diamine) promoted the dimerization/oligomerization of yeast IRE1 and concomitantly its RNase activity [37] , [38] , [40] , whereas compound 3 (1-(4-(8-amino-3-isopropylimidazo[1,5-a]pyrazin-1-yl)naphthalen-1-yl)-3-(3-(trifluoromethyl)phenyl)urea) inhibited the dimerization/oligomerization of human IRE1α and concomitantly its RNase function [39] . We posit that the structure of murine IRE1α reported here and human IRE1α reported previously, which do not adopt the back-to-back dimer configuration reflective of the ‘RNase-active’ state, provides insight into how in general dimer-breaking agents might act. Contrary to the expectation based on its effect on yeast IRE1, we discovered that ADP is an inhibitor of both the RNase and dimer/oligomerization activities of murine IRE1α in vitro . As assessed by velocity analytical ultracentrifugation, in the absence of ADP, IRE1 undergoes concentration-dependent oligomerization ( Fig. 6a ). Addition of ADP ( Fig. 6a ) and JAK inhibitor I ( Fig. 6a ) antagonized and enhanced this behaviour, respectively (see Fig. 6b for chemical structures). Consistent with these effects on oligomerization, ADP inhibited (IC 50 =117 μM) and JAK inhibitor I activated (EC 50 =0.19 μM) murine IRE1α RNase function in vitro ( Fig. 6c,d ). JAK inhibitor I exerted its influence on yeast IRE1 by engaging the kinase-active site [40] , and consistent with a common site of action on murine IRE1α, JAK inhibitor I potently inhibited auto-kinase activity with an IC 50 of 1.1 μM ( Fig. 6e ). Supporting the notion that murine IRE1α samples the same back-to-back dimer and higher-order polymer configurations demonstrated for yeast IRE1, murine IRE1α oligomerization was similarly dependent on (1) the N-terminal region preceding the kinase domain ( Fig. 6a ), (2) the integrity of the back-to-back dimer interface as assessed by a Asp620Ala mutation ( Fig. 6a ) and (3) enzyme phosphorylation status ( Fig. 6a ). Confirming the predicted importance of the yeast IRE1 back-to-back dimer configuration for murine IRE1α RNase function, dimer interface mutations in murine as shown for yeast IRE1 (ref. 11 ) also perturbed the RNase but not the kinase functions of murine IRE1α ( Fig. 6f,g ). These findings demonstrated that many of the regulatory features discerned for yeast IRE1 were general to murine IRE1α with the exception of the specific response to ADP. The findings further suggested that the crystal structure of murine IRE1α bound to ADP might provide a useful platform to discern the basis by which dimer-breaking inhibitors of IRE1 RNase function act. 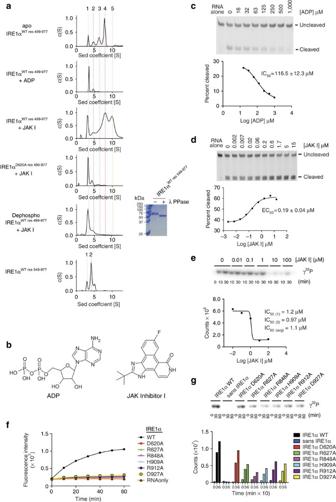Figure 6: Effects of kinase domain active site binders on murine IRE1α function. (a) Analysis of oligomerization status. Velocity analytical ultracentrifugation analyses were performed on murine IRE1α preparations (labelled on left) at 18 μM protein concentration. SeeSupplementary Fig. 6for full protein concentration series. ADP and JAK inhibitor I concentrations were 500 and 30 μM, respectively. SDS–PAGE analysis of murine IREα pre- and post-treatment with lambda phosphatase is shown in the right panel. (b) Chemical structures of ADP and JAK inhibitor I. (c) Effect of ADP on the RNase activity of murine IRE1α using a model single-hairpin substrate labelled with fluorescein. Reaction products were separated via PAGE, detected using a GE Healthcare Typhoon Variable Mode Imager (top panel) and quantified using ImageQuant 5 software (bottom panel). Shown is a representative profile. IC50±s.d. was calculated forn=3. (d) Dose-response analysis of JAK inhibitor I on the RNase activity of murine IRE1α assayed as inc. Shown is a representative profile. EC50±s.d. was calculated forn=3. (e) Dose-response analysis of JAK inhibitor I on the auto-kinase activity of murine IRE1α as assessed using P32-γ-ATP. Quantification plot presented in lower panel represents the 10 min time point from auto-radiographs in the top panel. Shown is a representative profile. IC50was calculated forn=2 (two experiments performed in singlicate). (f) Effect of the indicated back-to-back dimer interface mutations on murine IRE1α RNase function, as assayed inFig. 1b. (g) Effect of the indicated back-to-back dimer interface mutations on murine IRE1α auto-kinase function (phosphor image, top; quantification, bottom), as assayed inFig. 1c. Figure 6: Effects of kinase domain active site binders on murine IRE1α function. ( a ) Analysis of oligomerization status. Velocity analytical ultracentrifugation analyses were performed on murine IRE1α preparations (labelled on left) at 18 μM protein concentration. See Supplementary Fig. 6 for full protein concentration series. ADP and JAK inhibitor I concentrations were 500 and 30 μM, respectively. SDS–PAGE analysis of murine IREα pre- and post-treatment with lambda phosphatase is shown in the right panel. ( b ) Chemical structures of ADP and JAK inhibitor I. ( c ) Effect of ADP on the RNase activity of murine IRE1α using a model single-hairpin substrate labelled with fluorescein. Reaction products were separated via PAGE, detected using a GE Healthcare Typhoon Variable Mode Imager (top panel) and quantified using ImageQuant 5 software (bottom panel). Shown is a representative profile. IC 50 ±s.d. was calculated for n =3. ( d ) Dose-response analysis of JAK inhibitor I on the RNase activity of murine IRE1α assayed as in c . Shown is a representative profile. EC 50 ±s.d. was calculated for n =3. ( e ) Dose-response analysis of JAK inhibitor I on the auto-kinase activity of murine IRE1α as assessed using P 32 -γ-ATP. Quantification plot presented in lower panel represents the 10 min time point from auto-radiographs in the top panel. Shown is a representative profile. IC 50 was calculated for n =2 (two experiments performed in singlicate). ( f ) Effect of the indicated back-to-back dimer interface mutations on murine IRE1α RNase function, as assayed in Fig. 1b . ( g ) Effect of the indicated back-to-back dimer interface mutations on murine IRE1α auto-kinase function (phosphor image, top; quantification, bottom), as assayed in Fig. 1c . Full size image The kinase domain of murine IRE1α possessed a prototypical bilobal architecture consisting of an N-lobe rich in β-strands and a single regulatory helix αC, and a C-lobe composed predominantly of α-helices. In their active states, protein kinase domains can sample a closed conformation that aligns parallel regulatory and catalytic spines to productively bind and coordinate ATP within the inter-lobe cleft and to facilitate the phosphotransfer reaction [48] . The murine IRE1α kinase domain is notable in adopting a ‘kinase-inactive’ conformation in which the catalytic spine is intact but the regulatory spine is disrupted ( Fig. 7a , left panel). The catalytic spine, consisting of N-lobe residues Val586, Ala597 and the adenine ring of ADP, and C-lobe residues Leu649, Ile694, Leu695, Leu696, Val763 and Val767, forms a continuous hydrophobic column that spans the vertical length of the kinase domain. The regulatory spine in contrast, consisting of the N-lobe residues Leu616 and Tyr628 and the C-lobe residues His686 and Phe712, forms a broken hydrophobic column partitioned midway by a mispositioned Leu616 side chain, which projects from a non-productive, laterally displaced helix αC. A non-productive orientation of helix αC also manifests a loss of the ATP-coordinating salt bridge between the kinase domain invariant residues Lys599 (subdomain II) and Glu612 (subdomain III). Specifically, a 9-Å lateral shift of Glu612 prohibited the close ( ≅ 3.5 Å) interaction with Lys599 observed for the corresponding residues in yeast ‘kinase-active’ IRE1 structures ( Fig. 7b ). These two non-productive features of the murine IRE1α kinase domain are shared with the human IRE1α kinase domain structure also bound to ADP [46] , and differ from all yeast IRE1 co-structures bound to dimer promoting small molecule effectors ( Fig. 7a , right panel). 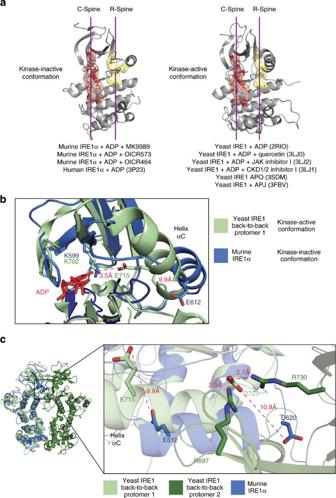Figure 7: Structure analysis of the kinase domain of murine IRE1α. (a) Ribbons’ representation of IRE1α kinase domains highlighting regulatory (yellow) and catalytic (red) spine alignments. All yeast structures solved to date display productive alignment of spines (right), while HAA-bound murine IRE1α structures and the dephospho-human IRE1α structure adopt non-productive alignments of the regulatory spine. PDB code and the respective ligand engaging the kinase-active site are indicated. (b) Zoom-in view of the kinase-active site of murine IRE1α superimposed on yeast IRE1 (PDB 2RIO) highlighting the displaced position of helix αC. (c) Zoom-in view of the projected back-to-back dimer interface of murine IRE1α (only one protomer shown) superimposed on the yeast IRE1 back-to-back dimer (PDB 2RIO) highlighting the physical link between helix αC and the back-to-back dimer interface. Side chains composing an essential intra-dimer salt bridge and the subdomain III glutamate side chain are shown as sticks. Figure 7: Structure analysis of the kinase domain of murine IRE1α. ( a ) Ribbons’ representation of IRE1α kinase domains highlighting regulatory (yellow) and catalytic (red) spine alignments. All yeast structures solved to date display productive alignment of spines (right), while HAA-bound murine IRE1α structures and the dephospho-human IRE1α structure adopt non-productive alignments of the regulatory spine. PDB code and the respective ligand engaging the kinase-active site are indicated. ( b ) Zoom-in view of the kinase-active site of murine IRE1α superimposed on yeast IRE1 (PDB 2RIO) highlighting the displaced position of helix αC. ( c ) Zoom-in view of the projected back-to-back dimer interface of murine IRE1α (only one protomer shown) superimposed on the yeast IRE1 back-to-back dimer (PDB 2RIO) highlighting the physical link between helix αC and the back-to-back dimer interface. Side chains composing an essential intra-dimer salt bridge and the subdomain III glutamate side chain are shown as sticks. Full size image The non-productive orientation of helix αC is notable as helix αC forms an integral component of the back-to-back dimer interface of ‘RNase-active’ yeast IRE1 structures [11] , [37] and may provide a link between ligand binding to the kinase-active site and back-to-back dimerization. IRE1-invariant residues Arg697, Asp723 and Arg730 in yeast IRE1 (corresponding to Arg594, Asp620 and Arg627 in murine IRE1α) form an essential three-centre salt bridge across the back-to-back dimer interface ( Fig. 7c ) that is required for the RNase function of both yeast [11] and murine ( Fig. 6f ) enzymes. In the murine IRE1α structure, the lateral shift in helix αC displaces Asp620 10.8 Å from the required position to interact with Arg594 and Arg627 ( Fig. 7c ). Since the three-centre intermolecular salt bridge is essential for the back-to-back dimerization and RNase function of murine IRE1α ( Fig. 6a,f ), we reason that the non-productive conformation of helix αC is responsible for the decreased propensity of murine IRE1α to adopt the back-to-back dimer configuration when bound to ADP. Our studies reveal how HAA inhibitors engage the RNase-active site of IRE1α with high affinity and specificity by exploiting a shallow complementary pocket and an essential Schiff base interaction between the aldehyde moiety of the inhibitor and the side chain amino group of Lys907. The presented HAA co-structures allow for a rationalization of current SAR and provide a platform for further rounds of optimization to improve inhibitor potency, bioavailability and selectivity. Interestingly, despite the fact that the HAA contact residues in IRE1α are highly conserved, yeast IRE1 is relatively resistant (~100-fold) to the fused dual-ring core of MKC9989, whereas it is equally sensitive to the single-ring core of OICR464 and OIRC573. This trend holds true also for the fused dual-ring core of the naphthalene scaffold ( Fig. 5 , first panel). As only a conservative substitution of Phe889 to tyrosine in yeast IRE1 differentiates the respective HAA-binding pockets, we speculate that this behaviour may be due to differences in binding pocket plasticity, which may be less accommodating for chemical scaffolds employing planar dual-ring cores in yeast IRE1. As IRE1α and β human isoforms are 100% identical in the composition of HAA-binding pocket residues ( Supplementary Fig. 4 ), we anticipate that both isoforms will be sensitive to inhibition by HAA inhibitors, although our findings with yeast IRE1 hold out the possibility for isoform selectivity despite similarities in binding pocket composition. The observation that HAA inhibitors centrally engage the RNase-active site by exploiting three of four invariant and essential catalytic residues for binding would explain their general effectiveness against both XBP1 splicing and RIDD cleavage targets [41] , [43] . The exploitation of essential catalytic residues for binding may also impose a major impediment to the acquisition of resistance mutations if employed in a clinical setting, since mutations shown here that abrogate HAA binding also compromise IRE1α RNase catalytic activity. Finally, RNase L, the sole paralogue of IRE1α in mammals, notably lacks an appropriately positioned lysine residue for Schiff base formation (substituted for leucine in human RNase L) and shares only three of eight other contact residues (equivalent to the invariant catalytic residues Tyr892, Asn906 and His910 in human IRE1α). These differences likely account for the observed resistance of RNase L to HAA inhibitors [41] , [43] . Although the core scaffold and ring substituents of MKC9989 make no overt clash with RNA, substitutions at position 3 with far bulkier groups have great potential to hinder RNA binding through clashes with the scissile phosphate group. Such substitutions would be expected to cause a transition of an HAA analogue from a substrate non-competitive to a substrate competitive mechanism of action. We speculate that elaboration of HAA inhibitor structure to exploit the RNA substrate-binding infrastructure (for example, by covalently linking an HAA to a dinucleotide mimetic), to impart a competitive mechanism of action, may also provide a means to improve inhibitor potency further. By capturing favourable or disfavourable interactions with specific RNA substrates, it may also be possible to engineer HAA analogues with inhibitory properties that discriminate between the numerous XBP1 and RIDD substrates. Small molecule binders to the kinase domain of IRE1 that support a non-productive outwardly displaced conformation of helix αC, as promoted by ADP in the human and mouse IRE1α crystal structures, will function as protein kinase inhibitors by virtue of competitively inhibiting ATP binding, but might also function as RNase inhibitors by preventing attainment of the productive back-to-back dimer configuration required for RNase activity. As such, the crystal structures of mouse and human IRE1α would provide useful platforms for the design of small molecule kinase inhibitors that repress RNase function. Towards this end, we speculate that compound 3 (1-(4-(8-amino-3-isopropylimidazo[1,5-a]pyrazin-1-yl)naphthalen-1-yl)-3-(3-(trifluoromethyl)phenyl)urea), a first in class ATP-competitive protein kinase inhibitor that inhibits IRE1 RNase function [39] , might act through such a mechanism. Biomolecules containing aldehyde moieties are common in both food stuffs, essential nutrients and vitamins, including vanilla, sugars (glucose) and vitamins A and B 6 . Although some aldehyde-containing compounds can form irreversible adducts, this is limited to unsaturated hydroxylated aliphatic chains such as lipid peroxidation products including 4-hydroxynonenal, which can induce ER stress [49] , or hydroxylated saturated aliphatic chains where an Amadori rearrangement is required after the imine is formed. This is the case of HbA1c generation by glucose on haemoglobin [50] , the major biomarker of long-term glucose exposure in diabetics. Aromatic aldehydes including pyridoxal phosphate (vitamin B 6 ) are unable to undergo such conversion. Furthermore, Schiff bases are not stable in the presence of water and studies indicate that dissociation from the mammalian IRE1α is rapid both on the enzyme in vitro and in cells after washout [41] , [43] . Therefore, stable adduct formation and creation of new epitopes by lysine conversion are not likely for IRE1 or other proteins limiting the possibility of immune recognition and sensitization in vivo ; however, transient adduct formation of buried lysines in heterologous enzymes cannot be formally ruled out. HAA compounds designed to enhance the oxygen saturation of haemoglobin have long serum half-lives and excellent target-binding properties in humans [51] , contrary to conventional wisdom. Indeed, HAA inhibitors of IRE1α are active and well-tolerated in vivo ; first, the biphenyl HAA analogue, compound 2, synergized with an oncolytic virus [44] , second, the naphthalene compound MKC3946 was readily tolerated with high exposure where it inhibited the splicing of XBP1 mRNA in tissues and tumours and reduced myeloma tumour growth [42] and finally, the coumarin compound 4μ8C was effective in suppressing XBP1s, inflammatory cytokines and inflammation in a rheumatoid arthritis model [52] . These studies suggest that HAA compounds may be highly selective for the RNase-active site of IRE1α and can be administered in vivo to obtain desired effects. XBP1 splicing and CD59 stability analysis Human RPMI 8226 plasmacytoma cells were grown in monolayer culture using Dulbecco’s modified Eagle’s medium supplemented with 10% fetal calf serum at 37 °C and 5% CO 2 . MKC9989 was prepared as 10 mM stocks in DMSO, stored at −20 °C and diluted in medium as indicated. Thapsigargin (Tg) was resuspended in DMSO and diluted in medium. Cells were grown to 50% confluency, treated with 1 μM Tg and/or 10 μM MKC9989 at the indicated time points. Following incubation of cells for the indicated periods, cells were collected. Procedures for preparation and measurement of XBP1s , XBP1u and CD59 mRNAs were as described previously [41] . Protein expression and purification Murine IRE1α residues 499–977 used for in vitro biochemical and biophysical analyses and IRE1α residues 549–977 used for X-ray crystallographic analyses, both harbouring an Asn772Tyr substitution, were expressed in SF9 insect cells using the Bac-to-Bac baculovirus system (Invitrogen). IRE1α fragments were cloned into pFastBac HTA vector as N-terminal polyhistidine tag fusions and viruses were generated according to manufacturer’s instructions. Large-scale protein expression was performed from 8 l cultures of SF9 cells grown in suspension. Following 3 days post infection, cells were collected by centrifugation, lysed by sonication in lysis buffer containing: 0.1 M Tris pH 7.0, 1 M NaCl, 25 mM imidazole, 1 mM tris (2-carboxyethyl) phosphine (TCEP) and 10% glycerol, and purified by Ni immobilized-metal affinity chromatography. The polyhistidine tag was cleaved with Tobacco etch virus protease and subtracted by an additional immobilized-metal affinity chromatography step. Following size-exclusion chromatography using a Superdex S200 column equilibrated in 25 mM Hepes pH 7.0, 0.5 M NaCl and 2 mM TCEP, pure fractions were pooled and concentrated to 10 mg ml −1 and flash frozen in liquid nitrogen. Human IRE1α residues 462–977 and yeast IRE1 residues 658–1,115 (with an internal deletion from Cys869 to Phe892) were expressed and purified as described previously [11] , [41] . In brief, yeast IRE1 was expressed from a pProEX plasmid in Escherichia coli BL21 cells as a polyhistidine-tagged fusion. Human IRE1α was expressed using the Bac-N-Blue baculovirus system and SF9 insect cells as a GST-tagged fusion. Proteins were purified using Ni-nitrilotriacetic acid (NTA) and glutathione resin chromatography, respectively, followed by protease cleavage of the affinity tag and finally by size-exclusion chromatography on a Superdex S200 column. Crystallization and structure determination Complexes were preformed on ice for 30 min before crystallization. The final solution contained 200 μM IRE1α, 1 mM inhibitor, 0.5% DMSO (v/v), 2 mM ADP, 2 mM MgCl 2 , 2 mM TCEP, 25 mM HEPES, pH 7.0. Crystals were grown at 20 °C by mixing the preformed complex with precipitant solution containing 0.1 M HEPES, 12% PEG8000 and 8% ethylene glycol at pH 7.5. Rod-shaped crystals ~0.15 mm in length grew after a week, and were flash frozen in liquid N 2 before data collection. All data sets were processed using XDS [53] . Anisotropic truncation and scaling was applied using the UCLA MBI Diffraction Anisotropy Server ( http://services.mbi.ucla.edu/anisoscale ) [54] . The structure of the IRE1α–MKC9989 complex was solved by molecular replacement using CCP4-PHASER [55] and the structure of human IRE1α (PDB 3P23 (ref. 46 )) as the search model. The other HAA complexes were solved using the IRE1α–MKC9989 structure as the search model. All structures were refined using PHENIX Refine [56] . Real space inspection and refinement was performed using COOT [57] . ADP, Mg 2+ and the inhibitors were manually positioned in difference maps. Geometric restraints for the inhibitors were generated using eLBOW (PHENIX package) [58] . All inhibitors that were modelled were covalently bound to the Lys907 through a Schiff base. For IRE1α-OICR573 and IRE1α-OICR464 structures, a long tubular density at the surface of one protein protomer was modelled as a PEG (polyethylene glycol) molecule. Data sets for MKC9989, OICR573 and OICR464 co-structures were collected at 100 K at 0.979 Å (NE-CAT beamline 24-ID-C), 1.540 Å (home source) and 0.979 Å wavelengths (NE-CAT beamline 24-ID-C), respectively. Ramachandran statistics corresponding to outliers, allowed and favoured regions for the MKC9989 co-structure were 0.79, 6.9 and 93.02%, for the OICR573 co-structure were 0.33, 4.09 and 95.58% and for the OICR464 co-structure were 0.47, 4.93 and 94.61%, respectively. In vitro kinase assays Auto-phosphorylation kinase assay in Fig. 6e was performed with 1.5 μM murine IRE1α and 150 μM ATP spiked with 27.7 nM P 32 -γ-ATP. Reactions were pre-incubated with IRE1α and inhibitor for 1 h at room temperature. After addition of ATP reaction mix, reactions were incubated at room temperature. Reactions were terminated by addition of SDS–polyacrylamide gel electrophoresis (PAGE) 6 × loading buffer and analysed by SDS–PAGE using NuPage 4–12% Bis-Tris gels. P 32 -γ-ATP signal was detected by phosphor imaging using a GE Healthcare Typhoon Variable Mode Imager. Quantification was performed using ImageQuant5 software. Trans auto-phosphorylation assays in Figs 1c , 4c and 6g were performed as above, except with 150 nM of IRE1α and 15 μM of kinase dead (Asp797Ala) yeast IRE1, residues 658–1115, as a phosphoacceptor substrate. Endoribonuclease assays Fluorescence-based RNA cleavage assays were performed with 10 nM IRE1α protein and 100 nM of a single hairpin RNA substrate (5′- CAUGUCCGCAGCGCAUG -3′), labelled on the 5′ and 3′ termini with Alexa Fluor 647 fluorophore and black hole quencher, respectively. Reaction buffer consisted of 50 mM Tris pH 7.0, 0.5 mM MgCl 2 , 10 mM KCl, 0.025% Tween-20, 0.063 mg ml −1 tRNA and 2 mM dithiothreitol. Compounds were pre-incubated in reaction buffer with IRE1α proteins for 1 h at room temperature. On addition of RNA substrate (diluted in 10 mM Tris pH 7.0 and 0.1 mM EDTA), cleavage reactions were monitored in real time by fluorescence intensity ( λ excited =651 nm, λ emission =672 nm) at 2-min intervals using a Molecular Dimensions Analyst HT microplate reader. Gel-based RNA cleavage assays were performed in the same reaction buffer as above with the addition of 0.09 mg ml −1 bovine serum albumin. A single hairpin RNA substrate (5′- CAUGUCCGCAGCGCAUG -3′) labelled with fluorescein on the 5′ terminus was used at a concentration of 45 nM. Reactions were pre-incubated with inhibitor compound for 1 h at room temperature, and then on addition of RNA substrate for 10–45 min at 37 °C. Reactions were quenched by addition of 2 × RNA loading buffer (90% (v/v) formamide, 25 mM EDTA) and samples were analysed using 20% Urea-TBE (Tris/Borate/EDTA) PAGE and imaged via a GE Healthcare Typhoon Variable Mode Imager. Images were quantified using ImageQuant5 software. The gel-based RNase cleavage assay shown in Fig. 4d was performed in a reaction buffer containing 1 M Hepes pH 7.0, 100 mM ADP, 100 mM MgCl 2 and100 mM TCEP, with 100 μM murine IRE1α and 60 μM of an unlabelled dual-hairpin RNA substrate encompassing human XBP1 nucleotide positions 426–490 generated by in vitro transcription reactions. Cleavage reactions were pre-incubated with compound for 30 min on ice and after addition of RNA substrate further for 45 min at room temperature. Reactions were quenched by the addition of 2 × RNA loading buffer (90% formamide, 25 mM EDTA, 0.02% xylene cyanol and 0.02% bromophenol blue) and samples were analysed using 20% Urea-TBE PAGE, stained with RedSafe dye and imaged via a GE Healthcare Typhoon Variable Mode Imager. Direct HAA inhibitor-binding analyses Microscale thermophoresis was performed with 500 nM murine IRE1α and 0.05% Pluronic in non-coated standard capillaries. The reactions were performed in a buffer containing 25 mM Hepes pH 7.0, 0.5 M NaCl and 2 mM TCEP. MKC9989, OICR464 and OICR573 inhibitor-binding reactions employed final DMSO concentrations of 1, 5 and 2%, respectively. All measurements were performed at 20% microscale thermophoresis power and 20% light-emitting diode power using the Monolith NT.LabelFree instrument (NanoTemper Technologies). Chemical synthesis MKC9989, OICR573, OICR464 and the napthalene analogue series shown in Fig. 5 were synthesized using methods described in WO 2011/127070 A2 (MKC9989) and WO2008/154484 A1 (OICR573 and OICR464) with commercially available chemical reagents. (7-Hydroxy-6-methoxy-3-(2-(2-methoxyethoxy)ethyl)-4-methyl-2-oxo-2H-chromene-8-carbaldehyde) was synthesized as shown in Scheme 1 . 2-Hydroxy-3-methoxy-5-(4-methyl-3,4-dihydro-2H-benzo[b][1,4]oxazin-7-yl)benzaldehyde and 4-hydroxy-5-methoxy-4′-morpholino-[1,1′-biphenyl]-3-carbaldehyde were synthesized as shown in Scheme 2 and 3 , respectively. Toluene-4-sulphonic acid 2-(2-methoxy-ethoxy)-ethyl ester. A mixture of 125 ml aqueous NaOH (2.38 g, 0.0595, mol) solution and 200 ml tetrahydrofuran (THF) 2-(2-methoxy-ethoxy)-ethanol (5 g, 0.042 mol) was cooled to 0 °C in a round bottom flask. A 200 ml THF solution of TsCl (7.38 g, 0.0388, mol) was added dropwise to the flask with stirring while keeping the inner temperature below 5 °C. After the addition, the reaction mixture was stirred at 0 °C–5 °C for additional 2 h. The reaction mixture was poured into a flask with 500 ml ice water. The resulting mixture was extracted with 150 ml DCM trice. The combined dichloromethane (DCM) solution was washed with water and brine, dried over Na 2 SO 4 and concentrated to afford a light yellow needle-like solid as the desired product (9.50 g, yield: 89%). 1 H NMR (400 MHz, CDCl 3 ): δ 7.79 (d, J =8.4 Hz, 2H, ArH), 7.33 (d, J =8.4 Hz, 2H, ArH), 4.16 (t, J =4.8 Hz, 2H, CH 2 ), 3.68 (t, J =4.8 Hz, 2H, CH 2 ), 3.58–3.56 (m, 2H, CH 2 ), 3.48–3.47 (m, 2H, CH 2 ), 3.34 (s, 3H, OCH 3 ), 2.44 (s, 3 H, ArCH 3 ). 2-[2-(2-Methoxy-ethoxy)-ethyl]-3-oxo-butyric acid ethyl ester. To a 25 ml dimethylformamide (DMF) suspension of NaH (0.992 g, 0.0248, mol) in a round bottom flask was added dropwise a 550 ml DME solution of acetyl ethylacetate (3.07 g, 0.0236, mol) at 0 °C. After the addition, the resulting mixture was stirred at 20 °C for 30 min. To the flask at 20 °C was added successively a solution of toluene-4-sulphonic acid 2-(2-methoxy-ethoxy)-ethyl ester (6.79 g, 0.0247, mmol) in 100 ml DME and NaI (3.72 g, 0.0248, mol) powder. The resulting mixture was stirred at 20 °C for 2 h untill seeing some precipitate formed. The mixture was then heated to 80 °C overnight under N 2 . Progress of the reaction was monitored by liquid chromatography mass spectrometry (LCMS) analysis. The reaction was completed in 16 h. After a filtration and removing the precipitate, the filtrate was collected and concentrated to a minimum volume. It was then diluted with H 2 O and acidified with 2 N HCl to pH=3, extracted with 100 ml DCM trice. The combined DCM solution was concentrated to a crude product that was purified by silica gel column (PE: EA=6:1) chromatography affording a light yellow oil (1.8 g, 32% yield) as the product 2-[2-(2-methoxy-ethoxy)-ethyl]-3-oxo-butyric acid ethyl ester. 1 H NMR (400 MHz, CDCl 3 ): δ 4.19–4.16 (m, 2H, CH 2 ), 4.12–4.10 (m, 1H, CH), 3.66 (m, 1H, CH), 3.52-3.48 (m, 6H, 3CH 2 ), 3.36 (s, 3H, OCH 3 ), 2.25 (s, 3H, COCH 3 ), 2.17–2.11 (m, 2H, CH 2 ), 1.49 (t, J =7.2 Hz, 3H, CH 3 ). 7-Hydroxy-6-methoxy-3-[2-(2-methoxy-ethoxy)-ethyl]-4-methyl-chromen-2-one. 2-[2-(2-Methoxy-ethoxy)-ethyl]-3-oxo-butyric acid ethyl ester (2.25 g, 0.0097, mol) and 2-hydroxyl-3-methoxyl-phenol (1.30 g, 0.0093, mol) were mixed with 200 ml H 3 PO 4 in a round bottom flask. The reaction mixture was stirred at 45 °C for 2 days. After the reaction was completed, the mixture was diluted with EA (100 ml) and poured into a flask with 1 l ice water. The resulting mixture was stirred for 15 min. After a filtration, the solid obtained was washed with cold saturated NaHCO 3 , brine and H 2 O successively. The solid was dried with toluene azeotropy distillation affording a light yellow solid as the product (1.25 g, 41% yield). 1 H NMR (400 MHz, DMSO-d6): δ 7.14 (s, 1H, ArH), 6.74 (s, 1H, ArH), 3.85 (s, 3H, CH 3 ), 3.49–3.47 (m, 4H, 2CH 2 ), 3.41-3.33 (m, 2H, CH 2 ), 3.20 (s, 3H, CH 3 ), 2.78 (t, J =7.2 Hz, 2H, CH 2 ), 2.40 (s, 3H, CH 3 ). MKC9989 (7-hydroxy-6-methoxy-3-(2-(2-methoxyethoxy)ethyl)-4-methyl-2-oxo-2H-chromene-8-carbaldehyde). 7-Hydroxy-6-methoxy-3-[2-(2-methoxy-ethoxy)-ethyl]-4-methyl-chromen-2-one (2.0 g, 0.0064, mol) and hexamethylenetetramine (HTMA) (3.65 g, 0.026 mol) were dissolved in 85 ml trifluoroacetic acid (TFA) in a round bottom flask. The reaction mixture was heated to 95 °C for 2 h. Progress. After the reaction was completed, the reaction mixture was concentrated. The residue was diluted with H 2 O, extracted with 100 ml DCM trice. The combined DCM solution was washed with cold saturated NaHCO 3 , brine, dried over Na 2 SO 4 and concentrated. The remaining residue was purified with a silica gel column (DCM: MeOH=100:1) chromatography affording 1.3 g of desired crude product. The product was further purified by recrystallization from EA, affording 7-hydroxy-6-methoxy-3-(2-(2-methoxyethoxy)ethyl)-4-methyl-2-oxo-2H-chromene-8-carbaldehyde (0.8 g, 37% yield) as a yellow solid. 1 H NMR (400 MHz, CDCl 3 ): δ p.p.m. 12.46 (s, 1H, OH), 10.66 (s, 1H, CHO), 7.30 (s, 1H, ArH), 4.01 (s, 3H, ArOCH 3 ), 3.72 (t, J =6.8 Hz, 2H, CH 2 ), 3.65–3.64 (m, 2H, CH 2 ), 3.56–3.55 (m, 2H, CH 2 ), 3.40 (s, 3H, OCH 3 ), 3.02 (t, J =6.8 Hz, 2H, CH 2 ), 2.49 (s, 3H, CH 3 ); LCMS [M+H] + =337.2; 13 C NMR (126 MHz, DMSO-d6) δ p.p.m. 192.40, 160.38, 154.10, 149.15, 147.63, 144.96, 120.01, 113.59, 111.65, 09/42, 71.79, 69.91, 68.94, 58.56, 56.99, 28.15, 15.86. 5-Bromo-3-methoxy-2-(methoxymethoxy)benzaldehyde. MOM-Cl (1.4 ml, 19 mmol) was added dropwise to a stirring mixture of 5-bromo-2-hydroxy-3-methoxybenzaldehyde (4.0 g, 17 mmol) and K 2 CO 3 (4.8 g, 35 mmol) in DMF (100 ml) at 0 °C. The reaction was allowed to warm to room temperature with stirring overnight. The reaction was quenched with a saturated NH 4 Cl solution and the product was extracted into EtOAc. The combined organic extracts were dried and concentrated to dryness in vaccuo . The residue was purified by flash chromatography (EtOAc/hexanes) to afford the title compound (2.5 g, 53% yield) as a solid. LCMS [M+H]+=275.1. OICR464 (2-hydroxy-3-methoxy-5-(4-methyl-3,4-dihydro-2H-benzo[b][1,4]oxazin-7-yl)benzaldehyde). A mixture of 5-bromo-3-methoxy-2-(methoxymethoxy)benzaldehyde (0.100 g, 0.36 mmol), (4-methyl-3,4-dihydro-2H-benzo[b][1,4]oxazin-7-yl)boronic acid (0.074 g, 0.38 mmol), Pd(PPh 3 ) 4 (0.013 g, 0.011 mmol) and Na 2 CO 3 (0.116 g, 1.1 mmol) in DMF (2 ml) and H 2 O (2 ml) was irradiated in the microwave to a temperature of 105 °C for 20 min. The reaction was partitioned between EtOAc and H 2 O and the layers were separated. The organic layer was washed with H 2 O, dried over magnesium sulphate and concentrated to dryness. The residue was dissolved in THF (10 ml) and treated with 3 M HCl (Aq.) (10 ml). THF was removed and the resultant acidic media was extracted with DCM. The organics were concentrated to dryness and the residue was purified by flash chromatography (2–8% MeOH/DCM) to afford the title compound (0.105 g, 96% yield) as a yellow solid. 1 H NMR (500 MHz, DMSO-d6) δ p.p.m. : 10.28 (s, 1H), 7.42–7.36 (m, 2H), 7.10 (dd, J =2.0, 8.3 Hz, 1H), 7.00 (d, J =1.8 Hz, 1H), 6.76 (d, J =8.4 Hz, 1H), 4.30–4.23 (m, 2H), 3.93 (s, 3H), 3.27–3.24 (m, 2H), 2.86 (s, 3H); LCMS [M+H]+=300.2; 13 C NMR (126 MHz, DMSO-d6) δ p.p.m. : 192.76, 150.16, 149.24, 144.62, 136.54, 131.91, 129.24, 122.88, 119.53, 117.23, 115.76, 113.58, 113.26, 64.99, 56.68, 48.90, 38.76. 5-Bromo-3-methoxy-2-(methoxymethoxy)benzaldehyde. MOM-Cl (1.4 mL, 19 mmol) was added dropwise to a stirring mixture of 5-bromo-2-hydroxy-3-methoxybenzaldehyde (4.0 g, 17 mmol) and K 2 CO 3 (4.8 g, 35 mmol) in DMF (100 mL) at 0 °C. The reaction was allowed to warm to room temperature with stirring overnight. The reaction was quenched with a saturated NH 4 Cl solution and the product was extracted into EtOAc. The combined organic extracts were dried and concentrated to dryness in vaccuo . The residue was purified by flash chromatography (EtOAc/hexanes) to afford the title compound (2.5 g, 53% yield) as a solid. LCMS [M+H]+=275.1. OICR573 (4-hydroxy-5-methoxy-4'-morpholino-[1,1'-biphenyl]-3-carbaldehyde). A mixture of 5-bromo-3-methoxy-2-(methoxymethoxy)benzaldehyde (0.104 g, 0.38 mmol), (4-methyl-3,4-dihydro-2H-benzo[b][1,4]oxazin-7-yl)boronic acid (0.114 g, 0.55 mmol), Pd(PPh 3 ) 4 (0.022 g, 0.019 mmol) and Na 2 CO 3 (0.190 g, 1.5 mmol) in DMF (2 ml) and H 2 O (2 ml) was irradiated in the microwave to a temperature of 110 °C for 30 min. The reaction was partitioned between EtOAc and H 2 O and the layers were separated. The organic layer was washed with H 2 O, dried over magnesium sulphate and concentrated to dryness. The residue was dissolved in THF (10 ml) and treated with 3 M HCl (Aq.) (10 ml). THF was removed and the resultant acidic media were extracted with DCM. The organics were concentrated to dryness and the residue was purified by flash chromatography (10–70% Hexane/EtOAc) to afford the title compound (0.087 g, 73% yield) as a yellow solid. 1 H NMR (500 MHz, DMSO-d6) δ p.p.m. 10.32 (s, 1H), 10.35-10.15 (bs, 1H), 7.56 (d, J =8.7 Hz, 2H), 7.46 (s, 2H), 7.02 (d, J =8.7, 2H), 3.95 (s, 3H), 3.85–3.70 (m, 4H), 3.25–3.10 (m, 4H); 13 C NMR (126 MHz, DMSO-d6) δ p.p.m. 192.54, 150.73, 150.06, 149.23, 131.91, 130.35, 127.31 (2C), 122.98, 117.27, 115.86, 115.74 (2C), 66.52 (2C), 56.70, 48.74 (2C); LCMS [M+H]+=314.1. MKC3946 (2-hydroxy-6-[5-(4-methyl-piperazine-1-carbonyl)-thiophen-2-yl]-naphthalene-1-carbaldehyde) was synthesized as shown in Scheme 4 . 6-Bromo-2-hydroxy-naphthalene-1-carbaldehyde. A solution of titanium tetrachloride (16.5 ml, 28.5 g, 150 mM) in methylene chloride (300 ml) was stirred under ice cooling in a 2 l three-necked flask, equipped with a thermometer, a dropping funnel and a gas outlet with a paraffin oil-filled bubbler. To the flask, dichloromethyl methyl ether (24.4 ml, 31 g, 270 mM) was added dropwise for 10 min resulting in a yellow solution. Then, a solution of 6-bromo-2-naphthol (20 g, 89.7 mM) in methylene chloride (300 ml) was added dropwise for 30 min whereupon the color of the mixture turned deep brownish-red and only a slight (3–4 °C) increase in the internal temperature was observed. Thereafter, the cooling batch was removed and the mixture was stirred at ambient temperature overnight. The next day, 1,000 ml of 1 N hydrochloric acid was added under ice cooling whereupon, during the first 10–15 min of the addition, extensive gas evolution was observed. After the addition was complete and the color of the mixture turned yellow, a small amount (0.78 g after drying) of a brick-red insoluble substance was filtered off. The aqueous layer was separated and extracted with methylene chloride (2 × 100 ml). The combined organic solutions were washed with 1 N hydrochloric acid (100 ml), then with brine (5 × 100 ml), dried over anhydrous MgSO 4 and evaporated to dryness. The brownish-yellow residue was triturated with diethyl ether; the yellow crystalline product was filtered off, washed with diethyl ether and dried over solid NaOH under reduced pressure as the desired product (16.95 g, 75.3%), m.p. 142–146 °C, 1 H NMR (400 MHz, DMSO-d6) δ ppm: 11.90 (s, 1H), 10.76 (s, 1H), 8.92 (d, J =9.3 Hz, 1H), 8.16 (d, J =2.0 Hz, 1H), 8.10 (d, J =9.3 Hz, 1H), 7.72 (dd, J =9.0, 2.3 Hz, 1H), 7.30 (d, J =9.0 Hz, 1H). This product is used in the next step without any further purification. 2-Hydroxy-6-(4,4,5,5-tetramethyl-[1,3,2]dioxaborolan-2-yl)-naphthalene-1-carbaldehyde. A mixture of 6-bromo-2-hydroxy-naphthalene-1-carbaldehyde (10.0 g, 39.8 mM), 1,4-dioxane (160 ml, distilled freshly from sodium metal, under nitrogen), bis(pinacolato)diborone (11.1 g, 43.8 mM), powdered potassium acetate (11.8 g, 120 mM) and palladium[1,1′-bis(diphenylphosphino)ferrocene]dichloride methylene chloride complex (3.9 g, 4.8 mM) was stirred at 80–85 °C under a slow stream of nitrogen for 4 h. After cooling, the insolubles were filtered off and washed with 1,4-dioxane. The solvent was evaporated and the dark brown residue was purified by chromatography over silica (200 g) using methylene chloride as eluent to yield the product (10.4 g, 87.6%) a yellow powder in 86% HPLC purity, m.p. 115–118 °C.The product can be further purified by recrystallization from sixfold (v/w) diisopropyl ether with final yield as 54%. 1 H NMR (400 MHz, CDCl3) δ p.p.m. : 13.23 (s, 1H), 10.82 (s, 1H), 8.33 (d, J =8.8 Hz, 1H), 8.29 (s, 1H), 8.02 (d, J =9.0 Hz, 1H), 7.98 (dd, J =8.5, 1.3 Hz, 1H), 7.13 (d, J =9.0 Hz, 1H), 1.39 (s, 12H). 5-Bromo-thiophene-2-carbonyl chloride. 5-Bromo-thiophene-2-carboxylic acid (9.09 g was dissolved in 100 ml thionyl chloride and the solution was refluxed for 1 h. After completion of the reaction, the excess of thionyl chloride was removed under reduced pressure. (9.60 g) Solid residue was obtained and used in the next step without further purification. (5-Bromo-thiophen-2-yl)-(4-methyl-piperazin-1-yl)-methanone. 1-Me-piperazine (4.27 g) and 5.54 g of DIPEA were dissolved in 80 ml of dry methylene chloride and the resulting solution was added dropwise at 0 °C to a solution of 9.60 g of 5-bromo-thiophene-2-carbonyl chloride in dry methylene chloride. The stirred solution was allowed to warm to room temperature and was washed with water. The organic phase was separated, dried and evaporated. The obtained 12.08 g of light brown oil was allowed to stand in the refrigerator overnight whereupon it solidified to a yellow-brownish solid (yield=98%). The product was used directly for the next step without further purification. 2-Hydroxy-6-[5-(4-methyl-piperazine-1-carbonyl)-thiophen-2-yl]-naphthalene-1-carbaldehyde. 2-Hydroxy-6-(4,4,5,5-tetramethyl-[1,3,2]dioxaborolan-2-yl)- naphthalene-1-carbaldehyde (5.50 g, 18.4 μmol), (5-bromo-thiophen-2-yl)- (4-methyl-piperazin-1-yl)-methanone (5.60 g, 19.3 μmol) and sodium carbonate (11.70 g) were dissolved in a mixture of 500 ml dimethylformamide (DMF) and 500 ml water. To this mixture was added 644 mg tetrakis(triphenylphosphino)-palladium. The reaction mixture was heated to 100 °C under nitrogen atmosphere. The progress was monitored by TLC. After 1 h, the reaction mixture was evaporated and the solid residues were partitioned between 400 ml water and 300 ml chloroform. The aqueous phase was extracted with additional 300 ml chloroform. The combined organic layer was dried over sodium sulfate. Evaporation of the solvent resulted in 7.00 g of a reddish powder, which was purified by flash column chromatography with chloroform as eluent. The isolated 6.88 g of crude material were suspended in ethanol and cooled to 0 °C. Saturated solution of HCl (70 ml) in ethyl acetate was added to the stirred suspension and was stirred overnight at room temperature. An additional portion of HCl/EtOAc was then added, the suspension was cooled again to 0 °C. The product was filtered off, washed with EtOAc and diethyl ether to yield a yellow powder (5.67 g, 74%) as the desired product. 1 H NMR (400 MHz, CDCl 3 ) δ p.p.m. : 13.13 (br. s, 1H), 10.82 (s, 1H), 8.37 (d, J =9.0 Hz, 1H), 7.97–8.05 (m, 2H), 7.86 (dd, J =8.8, 2.0 Hz, 1H), 7.30–7.35 (m, 2H), 7.19 (d, J =9.0 Hz, 1H), 3.78–3.88 (m, 4H), 2.45–2.55 (m, 4H), 2.35 (s, 3H). LCMS [M+H] + =381.1. MKC3987 (7-bromo-2-hydroxy-naphthalene-1-carbaldehyde). This compound was synthesized in a same manner as 6-bromo-2-hydroxy-naphthalene-1-carbaldehyde as shown in Scheme 4 using 7-bromo-naphthalen-2-ol as the starting material. 1 H NMR (400 MHz, CDCl 3 ) δ p.p.m. : 13.17 (s, 1H, OH), 10.73 (s, 1H, CHO), 8.49 (s, 1H, ArH), 7.93 (d, 1H, J =8.8 Hz, ArH), 7.66 (d, 1H, J =8.8 Hz, ArH), 7.53 (dd, 1H, J =0.8, 8.8 Hz, ArH), 7.15 (d, J =8.8 Hz, ArH); LCMS [M+H] + m/e: 251 (100%), 253 (100%). MKC4027 (2-hydroxy-7-[4-(4-methyl-piperazine-1-carbonyl)-phenyl]-naphthalene-1-carbaldehyde). This compound was synthesized in a similar manner as shown in Scheme 4 using 7-bromo-2-hydroxy-naphthalene-1-carbaldehyde to make the Suzuki coupling boronic ester 2-hydroxy-7-(4,4,5,5-tetramethyl-[1,3,2]dioxaborolan-2-yl) -naphthalene-1-carbaldehyde, which was then coupled with (4-bromo-phenyl)-(4-methyl-piperazin-1-yl)-methanone to form the target compound. 1 H NMR (400 MHz, CDCl 3 ) δ p.p.m. : 13.2 (s, 1H, OH), 10.90 (s, 1H, CHO), 8.52 (d, 1H, J=0.8 Hz, ArH), 8.01 (d, 1H, J=8.8 Hz, ArH), 7.88 (d, 1H, J =8.8 Hz, ArH), 7.75 (ddd, 2H, J =0.8, 0.8, 8.4 Hz, ArH), 7.66 (dd, 1H, J =0.8 Hz, ArH), 7.55 (ddd, 2H, J =0.8, 0.8, 8.4 Hz, ArH), 7.17 (d, 1H, J =8.8 Hz, ArH), 3.7 (br, 4H, -CH 2 ), 2.5 (br, 4H, -CH 2 ), 2.35 (s, 3H, -CH 3 ); LCMS [M+H] + m/e: 375 (100%). MKC3426 (2-hydroxy-3-methoxy-naphthalene-1-carbaldehyde). Commercially sourced from Ambinter (Cat. No. Amb18653768) or Aurora Fine Chemicals LLC (Cat. No. A07.180.446). MKC3437 (2-hydroxy-1-naphthylaldehyde). Commercially sourced from Sigma-Aldrich (Cat. No. H45353-25G). MKC3820 (2-hydroxy-1-acetonaphthylaldehyde). Commercially sourced from Sigma-Aldrich (Cat. No. 303054-25G). MKC3964 (1-naphthylaldehyde). Commercially sourced from Sigma-Aldrich (Cat. No. N109-2G-A). Modelling of the IRE1α–hydroxy–aryl–aldehyde–RNA substrate complex The tRNA splicing endonuclease in complex with RNA substrate (PDB 2GJW) [47] was used as a template to model RNA substrate concurrently bound to murine IRE1α and MKC9989 ( Supplementary Fig. 3e ) as performed previously for yeast IRE1 (ref. 11 ). In brief, the catalytic tetrad of the tRNA endonuclease (Tyr246, Ser258, His257 and Lys287) was superimposed manually onto the respective invariant catalytic tetrad (Tyr892, Asn906, His910 and Arg905) of mouse IRE1α. The two nucleotides flanking the scissile bond of the substrate RNA corresponding to chain E positions deoxy-uridine 14 and adenosine 15 were then excised and mutated to the IRE1α substrate consensus guanosine followed by cytosine. The full structure of IRE1α, dinucleotide and MKC9989 was then energy minimized using Refmac [59] , [60] . How to cite this article: Sanches, M. et al . Structure and mechanism of action of the hydroxy–aryl–aldehyde class of IRE1 endoribonuclease inhibitors. Nat. Commun. 5:4202 doi: 10.1038/ncomms5202 (2014). Accession codes : Final coordinates and structure factors for the IRE1α-MKC9989, IRE1α-OICR573 and IRE1α-OICR464 co-structures have been deposited to the PDB with the respective accession codes: 4PL3 , 4PL4 and 4PL5 . Synthesis of MKC9989 (7-hydroxy-6-methoxy-3-(2-(2-methoxye thoxy)ethyl)-4-methyl-2-oxo-2H-chromene-8-carbaldehyde). Synthesis of OICR464 (2-hydroxy-3-methoxy-5-(4-methyl-3,4- dihydro-2H-benzo[b][1,4]oxazin-7-yl)benzaldehyde). Synthesis of OICR573 (4-hydroxy-5-methoxy-4'-morpholino-[1,1'- biphenyl]-3-carbaldehyde). Synthesis of MKC3946 ( 2-Hydroxy-6-[5-(4-methyl-piperazine-1- carbonyl)-thiophen-2-yl]-naphthalene-1-carbaldehyde).